Selective escape of proteins from the mitochondria during mitophagy Mitophagy refers to the degradation of mitochondria by the autophagy system that is regulated by Parkin and PINK1, mutations in the genes for which have been linked to Parkinson’s disease. Here we show that certain mitochondrial outer membrane proteins, including FKBP38 and Bcl-2, translocate from the mitochondria to the endoplasmic reticulum (ER) during mitophagy, thereby escaping degradation by autophagosomes. This translocation depends on the ubiquitylation activity of Parkin and on microtubule polymerization. Photoconversion analysis confirmed that FKBP38 detected at the ER during mitophagy indeed represents preexisting protein transported from the mitochondria. The escape of FKBP38 and Bcl-2 from the mitochondria is determined by the number of basic amino acids in their COOH-terminal signal sequences. Furthermore, the translocation of FKBP38 is essential for the suppression of apoptosis during mitophagy. Our results thus show that not all mitochondrial proteins are degraded during mitophagy, with some proteins being evacuated to the ER to prevent unwanted apoptosis. Autophagy is a process for degradation of macromolecules and organelles in the cytoplasm of eukaryotic cells [1] . The degradation of mitochondria by this process is referred to as mitophagy [2] , [3] , [4] , [5] . When damaged mitochondria lose their membrane potential, undergo fission or fail to undergo fusion, they become segregated from the mitochondrial network [6] and are engulfed by autophagosomes. The resulting vesicles eventually fuse with lysosomes, and their contents are degraded by lysosomal proteases [7] , [8] . Mitophagy is regulated by Parkin (also known as PARK2) and PTEN-induced putative kinase protein 1 (PINK1, also known as PARK6), mutations in the genes for which have been linked to hereditary forms of Parkinson’s disease [9] , [10] . PINK1 is rapidly and constitutively degraded under steady-state conditions in normal mitochondria by presenilin-associated rhomboid-like protein, a rhomboid protease present in the mitochondrial inner membrane, whereas it is stabilized in response to the loss of membrane potential in damaged mitochondria [11] , [12] . Stabilized PINK1 recruits Parkin from the cytosol to depolarized mitochondria and phosphorylates it, resulting in activation of the ubiquitin ligase (E3) activity of Parkin [8] , [13] , [14] , [15] . Parkin then contributes to the widespread degradation of mitochondrial outer membrane proteins that is associated with mitophagy [16] , [17] . FKBP38 is a member of the FK506-binding protein (FKBP) family [18] , [19] . FKBP38 contains a transmembrane domain (TM) and a short juxtamembrane sequence at its COOH-terminus (hereafter referred to as CSS, for COOH-terminal signal sequence), and it localizes predominantly to the mitochondrial outer membrane [20] . We have previously shown that FKBP38 contributes to the localization of the antiapoptotic proteins Bcl-2 and Bcl-x L to the mitochondria and thereby inhibits apoptosis [21] . An increase in the intracellular concentration of free Ca 2+ results in the formation of a heterodimeric complex of calmodulin and FKBP38 that promotes the interaction of FKBP38 with Bcl-2 (ref. 22 ). We now show that, whereas many mitochondrial proteins are degraded by mitophagy, FKBP38 and Bcl-2 escape from such degradation as a result of their rapid translocation from the mitochondria to the endoplasmic reticulum (ER). The CSS of FKBP38 and Bcl-2 is necessary and sufficient for this translocation, and the number of basic amino acids in the CSS determines their fate during mitophagy. Furthermore, the translocation of FKBP38 is essential to prevent apoptosis during mitophagy. Our results suggest that mitophagy is not a non-selective process that results in the degradation of the entire organelle, but rather constitutes a system for selective degradation in association with a selective salvage system for certain proteins. FKBP38 and Bcl-2 are not degraded during mitophagy Given the mitochondrial localization of FKBP38 (ref. 21 ) and its association with the proteasome [23] , we hypothesized that FKBP38 might have a role in mitophagy. We therefore examined the abundance of mitochondrial proteins during mitophagy in mouse embryonic fibroblasts (MEFs). Given that MEFs do not express Parkin [13] , we infected the cells with a retrovirus encoding enhanced green fluorescent protein (EGFP)-tagged Parkin. Mitophagy was then induced by exposure of the MEFs to the mitochondrial uncoupler carbonyl cyanide m -chlorophenylhydrazone (CCCP) at 30 μM, which triggers mitochondrial depolarization. Immunoblot analysis of MEF lysates revealed that the abundance of mitochondrial proteins such as TOM40, Tim23 and cytochrome c decreased with time of exposure to CCCP ( Fig. 1a ; see Supplementary Fig. S1a ), suggesting that these mitochondrial proteins undergo degradation in association with mitophagy. Unexpectedly, however, the abundance of FKBP38 was not decreased after exposure of the cells to CCCP. Similar results were obtained with MEFs treated with paraquat ( Supplementary Fig. S1b ), which was also previously shown to induce mitophagy [8] . 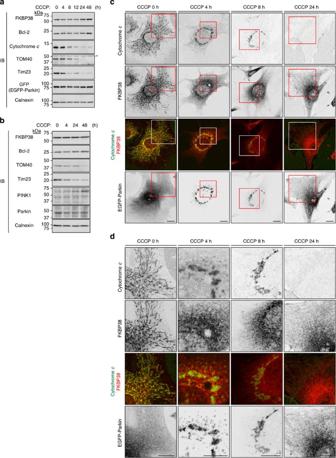Figure 1: FKBP38 is not degraded during mitophagy (a) MEFs stably expressing EGFP-Parkin were exposed to CCCP (30 μM) for the indicated times and then subjected to immunoblot analysis (IB) with antibodies to the indicated proteins. The asterisk indicates a nonspecific band. (b) SH-SY5Y cells were exposed to CCCP (10 μM) for the indicated times and then subjected to immunoblot analysis. (c) MEFs stably expressing EGFP-Parkin were treated with CCCP (30 μM) for the indicated times, fixed, permeabilized and subjected to immunofluorescence analysis with antibodies to FKBP38 and to cytochromecand with a confocal microscope. The fluorescence of EGFP-Parkin was monitored directly. (d) Higher-magnification views of the boxed areas inc. Scale bar (c,d), 10 μm. Figure 1: FKBP38 is not degraded during mitophagy ( a ) MEFs stably expressing EGFP-Parkin were exposed to CCCP (30 μM) for the indicated times and then subjected to immunoblot analysis (IB) with antibodies to the indicated proteins. The asterisk indicates a nonspecific band. ( b ) SH-SY5Y cells were exposed to CCCP (10 μM) for the indicated times and then subjected to immunoblot analysis. ( c ) MEFs stably expressing EGFP-Parkin were treated with CCCP (30 μM) for the indicated times, fixed, permeabilized and subjected to immunofluorescence analysis with antibodies to FKBP38 and to cytochrome c and with a confocal microscope. The fluorescence of EGFP-Parkin was monitored directly. ( d ) Higher-magnification views of the boxed areas in c . Scale bar ( c , d ), 10 μm. Full size image Given that FKBP38 associates with and determines the localization of Bcl-2 (ref. 21 ), we also examined the effect of CCCP on Bcl-2 abundance. Immunoblot analysis revealed that Bcl-2 was also resistant to degradation during mitophagy ( Fig. 1a ; Supplementary Fig. S1a,b ). To exclude the possibility that the resistance of FKBP38 and Bcl-2 to degradation during mitophagy reflects an artefact of Parkin overexpression in MEFs, we also monitored protein abundance in the human neuronal cell line SH-SY5Y, which expresses endogenous Parkin [24] . Exposure of SH-SY5Y cells to CCCP induced the rapid degradation of TOM40 and Tim23, whereas it did not affect the abundance of FKBP38 and Bcl-2 ( Fig. 1b ). These results suggested that not all mitochondrial proteins are necessarily degraded during mitophagy. We next examined the effect of CCCP on the subcellular localization of FKBP38 in MEFs expressing EGFP-Parkin. Immunofluorescence analysis revealed that cytochrome c and FKBP38 colocalized at the mitochondria in the absence of CCCP ( Fig. 1c ). (A quantitative analysis of these and subsequent immunofluorescence images is shown in Supplementary Fig. S2 .) At 4 h after the onset of CCCP exposure, mitochondria were aggregated around the nucleus and EGFP-Parkin was selectively recruited to the mitochondria. Consistent with the results of immunoblot analysis ( Fig. 1a ), signals for cytochrome c gradually decreased in intensity and had disappeared after exposure of the cells to CCCP for 24 h ( Fig. 1c ). In contrast, signals for FKBP38 remained after 24 h of CCCP treatment, but their initial tubular pattern indicative of a mitochondrial localization had changed to a fine meshwork pattern suggestive of localization to the ER. This shift in FKBP38 localization was detected as early as 4 h after the onset of CCCP treatment ( Fig. 1c ; see Supplementary Movie 1 ). Similar results were also obtained with cells treated with paraquat ( Supplementary Fig. S1c ). Immunofluorescence analysis with antibodies to ubiquitin revealed that ubiquitin was concentrated at the mitochondria during mitophagy, but that it did not colocalize with FKBP38 ( Supplementary Fig. S3a ). CCCP treatment of native MEFs (not expressing Parkin) resulted in a loss of mitochondrial membrane potential and fragmentation of mitochondria ( Supplementary Fig. S3b ), but it did not elicit mitophagy. FKBP38 colocalized with cytochrome c at 8 h after the onset of CCCP treatment in these cells, suggesting that the putative translocation of FKBP38 from the mitochondria to the ER is not the direct result of mitochondrial depolarization and that it requires the progression of Parkin-dependent mitophagy. Consistent with these observations, immunoblot analysis revealed that mitochondrial proteins such as TOM40, Tim23, cytochrome c , FKBP38 and Bcl-2 were not degraded in the absence of Parkin in MEFs exposed to CCCP ( Supplementary Fig. S3c ). We next examined whether autophagy induced by amino-acid deprivation affects the localization of FKBP38. Culture of MEFs in medium lacking amino acids for 4 h resulted in the conversion of cytosolic LC3 (LC3-I) to membrane-bound, phosphatidylethanolamine-conjugated LC3 (LC3-II), as well as in downregulation of the phosphorylation of ribosomal S6 kinase (S6K) at Thr 389 , suggesting that autophagy was indeed induced. The level of FKBP38 did not change during autophagy induced by amino-acid starvation, however ( Supplementary Fig. S3d ). Immunofluorescence analysis confirmed that EGFP-LC3-positive punctate structures representing isolation membranes and autophagosomes were formed in response to amino-acid deprivation for 2 h, whereas FKBP38 remained colocalized with cytochrome c at the mitochondria ( Supplementary Fig. S3e ). Together, these results suggested that the translocation of FKBP38 occurs specifically during mitophagy, not in response to the simple loss of mitochondrial membrane potential or during autophagy other than mitophagy. FKBP38 translocates to the ER during mitophagy We next examined in more detail the subcellular localization of FKBP38 after the induction of mitophagy. Given that FKBP38 immunoreactivity showed a meshwork-like pattern suggestive of ER localization during mitophagy, we first determined whether FKBP38 colocalizes with VAP-A, an ER-resident protein [25] , by infecting MEFs with retroviruses encoding FLAG epitope-tagged Parkin and EGFP-tagged VAP-A. In the absence of CCCP, FKBP38 localized to the mitochondria and did not colocalize with EGFP-VAP-A ( Fig. 2a ). Treatment of the cells with CCCP for 24 h, however, resulted in the almost complete colocalization of FKBP38 with EGFP-VAP-A. Exposure of MEFs to Bafilomycin A1, which inhibits lysosomal activity, did not affect the CCCP-induced translocation of FKBP38 ( Supplementary Fig. S4 ), suggesting that the translocation is independent of lysosomal activity. The colocalization of FKBP38 with haemagglutinin epitope (HA)-tagged VAP-A was also observed in HeLa cells coexpressing FLAG-Parkin and treated with CCCP for 4 h ( Fig. 2c ). 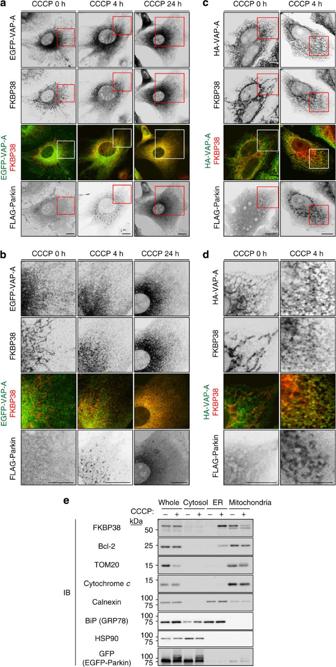Figure 2: FKBP38 translocates from the mitochondria to the ER during mitophagy. (a,c) MEFs (a) or HeLa cells (c) stably expressing FLAG-Parkin and either EGFP-VAP-A or HA-VAP-A were treated with CCCP (30 and 10 μM, respectively) for the indicated times, fixed, permeabilized and subjected to immunofluorescence analysis with antibodies to FKBP38, to HA or to FLAG (M2). The fluorescence of EGFP-VAP-A was also monitored directly. (b,d) Higher-magnification views of the boxed areas inaandc, respectively. (e) NIH 3T3 cells stably expressing EGFP-Parkin were incubated in the absence or presence of CCCP (30 μM) for 4 h, after which whole-cell homogenates as well as cytosolic, ER and mitochondrial fractions were prepared and subjected to immunoblot analysis. Scale bar (a–d), 10 μm. Figure 2: FKBP38 translocates from the mitochondria to the ER during mitophagy. ( a , c ) MEFs ( a ) or HeLa cells ( c ) stably expressing FLAG-Parkin and either EGFP-VAP-A or HA-VAP-A were treated with CCCP (30 and 10 μM, respectively) for the indicated times, fixed, permeabilized and subjected to immunofluorescence analysis with antibodies to FKBP38, to HA or to FLAG (M2). The fluorescence of EGFP-VAP-A was also monitored directly. ( b , d ) Higher-magnification views of the boxed areas in a and c , respectively. ( e ) NIH 3T3 cells stably expressing EGFP-Parkin were incubated in the absence or presence of CCCP (30 μM) for 4 h, after which whole-cell homogenates as well as cytosolic, ER and mitochondrial fractions were prepared and subjected to immunoblot analysis. Scale bar ( a – d ), 10 μm. Full size image To confirm further the translocation of FKBP38 from the mitochondria to the ER, we performed subfractionation of NIH 3T3 cells expressing EGFP-Parkin and treated with CCCP for 4 h. Immunoblot analysis of the fractions revealed that FKBP38 disappeared from the mitochondrial fraction and concomitantly appeared in the ER fraction in response to CCCP treatment ( Fig. 2e ). In contrast, subcellular localization of the mitochondrial markers cytochrome c and TOM20 as well as that of the ER markers BiP (GRP78) and calnexin did not change after exposure of the cells to CCCP. Collectively, the results of our immunofluorescence and subfractionation experiments indicated that FKBP38 indeed translocates from the mitochondria to the ER, and is thereby spared from degradation, during mitophagy. FKBP38 translocation requires Parkin but not proteasome RNA interference-mediated depletion of endogenous Parkin in SH-SY5Y cells inhibited the progression of mitophagy as well as FKBP38 translocation ( Supplementary Fig. S5 ). We next examined whether the E3 activity of Parkin is also required for FKBP38 translocation. A mutation (T240R) in the RING1 domain of Parkin abolishes the E3 activity of the protein [13] , [26] . Treatment with CCCP for 24 h induced neither mitophagy nor FKBP38 translocation in MEFs expressing EGFP-Parkin(T240R), whereas cytochrome c was degraded and FKBP38 translocated to the ER in those expressing wild-type EGFP-Parkin ( Fig. 3a ). Immunoblot analysis also revealed that cytochrome c was not degraded in response to CCCP treatment in cells expressing EGFP-Parkin(T240R) ( Fig. 3b ). These results thus showed that the E3 activity of Parkin is directly or indirectly required for FKBP38 translocation from the mitochondria to the ER during mitophagy. 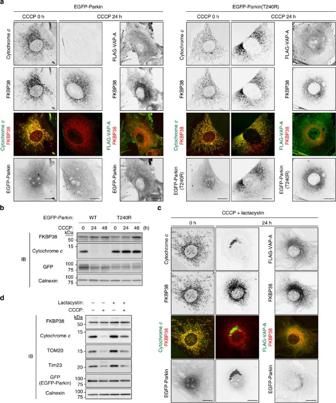Figure 3: FKBP38 translocation requires the E3 ligase activity of Parkin but not proteasome activity. (a) MEFs stably expressing EGFP-tagged wild-type (WT) or T240R mutant forms of Parkin as well as FLAG-tagged VAP-A were incubated in the absence or presence of CCCP (30 μM) for 24 h, fixed, permeabilized and subjected to immunofluorescence analysis with antibodies to FKBP38, to FLAG (M2) and to cytochromec. The fluorescence of EGFP was also monitored directly. (b) MEFs as inawere treated with CCCP (30 μM) for the indicated times and then subjected to immunoblot analysis. (c) MEFs stably expressing EGFP-Parkin and FLAG-VAP-A were incubated in the absence or presence of CCCP (30 μM) and lactacystin (10 μM) for 24 h, fixed, permeabilized and subjected to immunofluorescence analysis with antibodies to FKBP38, to FLAG (M2) and to cytochromec. The fluorescence of EGFP-Parkin was also monitored directly. (d) MEFs stably expressing EGFP-Parkin were incubated for 12 h in the absence or presence of CCCP (30 μM) and lactacystin (10 μM) as indicated and then subjected to immunoblot analysis. Scale bar (a,c), 10 μm. Figure 3: FKBP38 translocation requires the E3 ligase activity of Parkin but not proteasome activity. ( a ) MEFs stably expressing EGFP-tagged wild-type (WT) or T240R mutant forms of Parkin as well as FLAG-tagged VAP-A were incubated in the absence or presence of CCCP (30 μM) for 24 h, fixed, permeabilized and subjected to immunofluorescence analysis with antibodies to FKBP38, to FLAG (M2) and to cytochrome c . The fluorescence of EGFP was also monitored directly. ( b ) MEFs as in a were treated with CCCP (30 μM) for the indicated times and then subjected to immunoblot analysis. ( c ) MEFs stably expressing EGFP-Parkin and FLAG-VAP-A were incubated in the absence or presence of CCCP (30 μM) and lactacystin (10 μM) for 24 h, fixed, permeabilized and subjected to immunofluorescence analysis with antibodies to FKBP38, to FLAG (M2) and to cytochrome c . The fluorescence of EGFP-Parkin was also monitored directly. ( d ) MEFs stably expressing EGFP-Parkin were incubated for 12 h in the absence or presence of CCCP (30 μM) and lactacystin (10 μM) as indicated and then subjected to immunoblot analysis. Scale bar ( a , c ), 10 μm. Full size image We also examined whether proteasome activity affects the localization of FKBP38. Parkin-dependent degradation of dysfunctional mitochondria requires the autophagy system but not the proteasome. Under normal conditions, the proteasome is present in both the nucleus and cytoplasm of cells. However, CCCP was found to induce translocation of the proteasome to the perinuclear region, where it colocalized with aggregated mitochondria, in MEFs expressing Parkin [17] . Although the proteasome is required for degradation of mitochondrial outer membrane proteins associated with mitophagy, proteasome inhibition suppresses outer membrane rupture but not mitophagy. We therefore examined whether proteasome activity is required for the translocation of FKBP38 from the mitochondria to the ER. MEFs expressing EGFP-Parkin were treated with CCCP in the absence or presence of the proteasome inhibitor lactacystin. Lactacystin slowed the rate of mitophagy progression. Cytochrome c was thus still concentrated in the perinuclear region at 24 h after CCCP exposure, whereas FKBP38 had already translocated to the ER and did not colocalize with cytochrome c at this time ( Fig. 3c ). Consistent with these immunofluorescence data, immunoblot analysis revealed that cytochrome c , TOM20 and Tim23 were degraded after treatment with CCCP for 12 h and that such degradation was attenuated slightly by lactacystin, whereas FKBP38 was not degraded at this time in the presence of CCCP ( Fig. 3d ). Although lactacystin slowed the progression of mitophagy, mitochondria eventually disappeared after treatment with CCCP in the presence of the proteasome inhibitor (data not shown). We thus concluded that FKBP38 translocation is independent of proteasome activity. COOH-terminal domains of FKBP38 are integral to the escape We next investigated which domains of FKBP38 contribute to translocation by generating chimeric proteins of FKBP38 and Omp25, both of which reside in the mitochondrial outer membrane and expose their NH 2 - and COOH-termini to the cytosol and mitochondrial intermembrane space, respectively [27] ( Fig. 4a ). Omp25 did not undergo translocation but rather was degraded during mitophagy ( Fig. 4b ). The COOH-terminal domains (TM and CSS) of FKBP38 and Omp25 were swapped to yield two reciprocally chimeric proteins, FKBP38/Omp25 and Omp25/FKBP38 ( Fig. 4a ). We then compared the behaviour of EGFP-tagged forms of FKBP38, Omp25, FKBP38/Omp25 and Omp25/FKBP38 during mitophagy in MEFs expressing FLAG-Parkin by immunofluorescence analysis. In the absence of CCCP, all these proteins colocalized with the mitochondrial marker MitoTracker ( Supplementary Fig. S6a ). CCCP treatment for 4 h induced the translocation of FKBP38 and, to a lesser extent, that of Omp25/FKBP38 from the mitochondria to the ER ( Fig. 4b ; Supplementary Fig. S6b ). In contrast, Omp25 and FKBP38/Omp25 colocalized with cytochrome c after exposure of the cells to CCCP. Although Omp25 and FKBP38/Omp25 were almost completely degraded 24 h after exposure of the cells to CCCP, a substantial proportion of both FKBP38 and Omp25/FKBP38 remained at this time ( Fig. 4c ). These results suggested that the COOH-terminal domains of FKBP38 are necessary and sufficient for its translocation from the mitochondria to the ER during mitophagy. 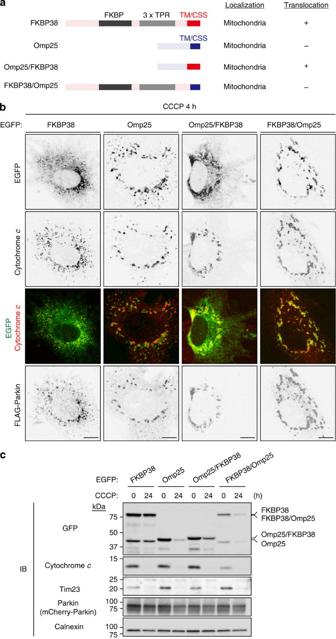Figure 4: FKBP38 translocation depends on its COOH-terminal domains. (a) Domain organization of FKBP38, Omp25 and the chimeric proteins Omp25/FKBP38 and FKBP38/Omp25, as well as a summary of their localization and ability to undergo translocation during mitophagy as determined in (b). (b) MEFs stably expressing FLAG-Parkin and EGFP-tagged forms of FKBP38, Omp25, Omp25/FKBP38 or FKBP38/Omp25 were treated with CCCP (30 μM) for 4 h, fixed, permeabilized and subjected to immunofluorescence analysis with antibodies to cytochromecand to FLAG (rabbit polyclonal). The fluorescence of EGFP was also monitored directly. Scale bar, 10 μm. (c) MEFs stably expressing mCherry-tagged Parkin and EGFP-tagged forms of FKBP38, Omp25, Omp25/FKBP38 or FKBP38/Omp25 were incubated in the absence or presence of CCCP (30 μM) for 24 h and then subjected to immunoblot analysis. Figure 4: FKBP38 translocation depends on its COOH-terminal domains. ( a ) Domain organization of FKBP38, Omp25 and the chimeric proteins Omp25/FKBP38 and FKBP38/Omp25, as well as a summary of their localization and ability to undergo translocation during mitophagy as determined in ( b ). ( b ) MEFs stably expressing FLAG-Parkin and EGFP-tagged forms of FKBP38, Omp25, Omp25/FKBP38 or FKBP38/Omp25 were treated with CCCP (30 μM) for 4 h, fixed, permeabilized and subjected to immunofluorescence analysis with antibodies to cytochrome c and to FLAG (rabbit polyclonal). The fluorescence of EGFP was also monitored directly. Scale bar, 10 μm. ( c ) MEFs stably expressing mCherry-tagged Parkin and EGFP-tagged forms of FKBP38, Omp25, Omp25/FKBP38 or FKBP38/Omp25 were incubated in the absence or presence of CCCP (30 μM) for 24 h and then subjected to immunoblot analysis. Full size image Bcl-2, but not Bcl-x L , escapes to the ER during mitophagy Similar to FKBP38, we found that Bcl-2 is not subjected to degradation during mitophagy ( Fig. 1a ). We next examined whether Bcl-x L , an antiapoptotic member of the Bcl-2 family of proteins, also escapes from mitophagy. Despite the structural and functional similarities between Bcl-2 and Bcl-x L , we found that Bcl-x L or EGFP-Bcl-x L was degraded during mitophagy in MEFs coexpressing EGFP- or FLAG-tagged Parkin and treated with CCCP ( Fig. 5a ; Supplementary Fig. S7 ). The degradation of EGFP-Bcl-x L as well as that of cytochrome c and Tim23 in cells expressing EGFP-Bcl-x L or EGFP-Bcl-2 appeared moderately attenuated compared with the degradation of mitochondrial proteins in cells not forcibly expressing these constructs, probably because Bcl-2 and Bcl-x L partially antagonize the autophagic process [28] , [29] . We examined whether the COOH-terminal domains of Bcl-2 and Bcl-x L are responsible for their fates by generating the domain-swap mutants Bcl-2/x L (cytosolic domain of Bcl-2 fused with the TM and CSS of Bcl-x L ) and Bcl-x L /2 (cytosolic domain of Bcl-x L fused with the TM and CSS of Bcl-2) ( Fig. 5b ). Immunofluorescence analysis of MEFs expressing FLAG- or mCherry-tagged Parkin revealed that, whereas EGFP-tagged forms of Bcl-2, Bcl-x L , Bcl-2/x L and Bcl-x L /2 colocalized with cytochrome c in the absence of CCCP treatment, Bcl-2 and Bcl-x L /2 did not colocalize with cytochrome c at 4 h after the onset of such treatment ( Fig. 5c ; Supplementary Fig. S8 ). These results thus suggested that the COOH-terminal domains of Bcl-2 are necessary and sufficient for its translocation during mitophagy, as shown for FKBP38, and that the difference between the COOH-terminal domains of translocating proteins (FKBP38 and Bcl-2) and those of degraded proteins (Omp25 and Bcl-x L ) determines protein fate during mitophagy. 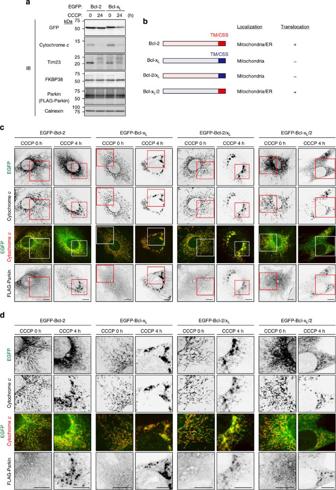Figure 5: Bcl-2 translocates from the mitochondria to the ER during mitophagy and Bcl-xLdoes not. (a) MEFs stably expressing FLAG-Parkin and either EGFP-Bcl-2 or EGFP-Bcl-xLwere incubated in the absence or presence of CCCP (30 μM) for 24 h and then subjected to immunoblot analysis. (b) Domain organization of Bcl-2, Bcl-xL, and the chimeric proteins Bcl-2/xLand Bcl-xL/2, as well as a summary of their localization and ability to translocate during mitophagy, as determined inc. (c) MEFs stably expressing FLAG-Parkin and EGFP-tagged forms of Bcl-2, Bcl-xL,Bcl-2/xLor Bcl-xL/2 were incubated in the absence or presence of CCCP (30 μM) for 4 h, fixed, permeabilized and subjected to immunofluorescence analysis with antibodies to cytochromecand to FLAG (rabbit polyclonal). The fluorescence of EGFP was also monitored directly. (d) Higher-magnification views of the boxed areas inc. Scale bar (c,d), 10 μm. Figure 5: Bcl-2 translocates from the mitochondria to the ER during mitophagy and Bcl-x L does not. ( a ) MEFs stably expressing FLAG-Parkin and either EGFP-Bcl-2 or EGFP-Bcl-x L were incubated in the absence or presence of CCCP (30 μM) for 24 h and then subjected to immunoblot analysis. ( b ) Domain organization of Bcl-2, Bcl-x L , and the chimeric proteins Bcl-2/x L and Bcl-x L /2, as well as a summary of their localization and ability to translocate during mitophagy, as determined in c . ( c ) MEFs stably expressing FLAG-Parkin and EGFP-tagged forms of Bcl-2, Bcl-x L, Bcl-2/x L or Bcl-x L /2 were incubated in the absence or presence of CCCP (30 μM) for 4 h, fixed, permeabilized and subjected to immunofluorescence analysis with antibodies to cytochrome c and to FLAG (rabbit polyclonal). The fluorescence of EGFP was also monitored directly. ( d ) Higher-magnification views of the boxed areas in c . Scale bar ( c , d ), 10 μm. Full size image Basicity of the CSS determines the escape of proteins The basicity of the CSS of Bcl-2 or Bcl-x L was previously shown to affect the localization of these proteins [30] . The CSS of each of the proteins shown to translocate from the mitochondria to the ER during mitophagy (FKBP38 and Bcl-2) contains only one strongly basic amino acid (arginine or lysine), whereas two or three such amino acids are present in the CSS of the degraded proteins Omp25 and Bcl-x L ( Fig. 6 ), suggesting that the basicity of the CSS might be a determinant of translocation. To test this possibility, we replaced the COOH-terminal asparagine of FKBP38 with lysine, yielding a mutant, FKBP38(N402K), whose CSS is more basic than that of wild-type FKBP38 ( Fig. 6 ). Immunofluorescence analysis of MEFs coexpressing FLAG-Parkin revealed that EGFP-FKBP38(N402K) largely colocalized with cytochrome c ; it did not colocalize with wild-type FKBP38 tagged with mCherry at 4 h after exposure of the cells to CCCP ( Fig. 7a ; see also Supplementary Fig. S9a ). Immunoblot analysis further showed that the mutant protein had been degraded to a greater extent than EGFP-FKBP38 after CCCP treatment for 24 h ( Fig. 7c ). We performed similar experiments with the mutant Bcl-2(H235R), in which a histidine in the CSS of Bcl-2 was replaced with arginine ( Fig. 6 ). This mutant was also defective in translocation from the mitochondria to the ER during mitophagy ( Fig. 7e ; Supplementary Fig. S9b ). 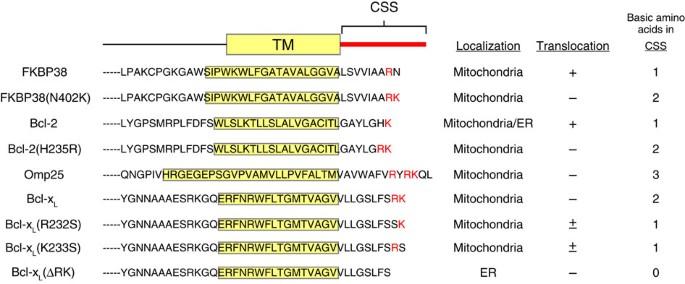Figure 6: COOH-terminal signal sequences of wild-type and mutant mitochondrial proteins. The structure of the CSS as well as a summary of the subcellular localization, ability to translocate during mitophagy and number of basic amino acids in the CSS are shown for each protein. Figure 6: COOH-terminal signal sequences of wild-type and mutant mitochondrial proteins. The structure of the CSS as well as a summary of the subcellular localization, ability to translocate during mitophagy and number of basic amino acids in the CSS are shown for each protein. 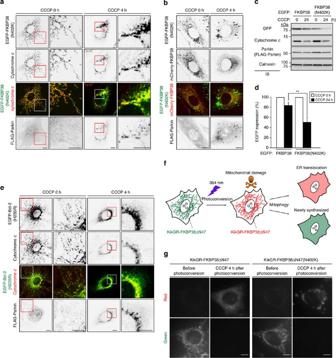Figure 7: Basic residues in the CSS determine protein translocation during mitophagy. (a) MEFs stably expressing EGFP-FKBP38(N402K) and FLAG-Parkin were incubated in the absence or presence of CCCP (30 μM) for 4 h, fixed, permeabilized and subjected to immunofluorescence analysis with antibodies to cytochromecand to FLAG (rabbit polyclonal). The fluorescence of EGFP-FKBP38(N402K) was also monitored directly. Higher-magnification views of the boxed areas are shown in the right panels of each set. (b) MEFs stably expressing EGFP-FKBP38(N402K), mCherry-FKBP38 and FLAG-Parkin were incubated in the absence or presence of CCCP (30 μM) for 4 h, fixed, permeabilized and subjected to immunofluorescence analysis with antibodies to FLAG (M2). The fluorescence of EGFP-FKBP38(N402K) and mCherry-FKBP38 was also monitored directly. (c) MEFs stably expressing FLAG-Parkin and either EGFP-FKBP38 or EGFP-FKBP38(N402K) were incubated in the absence or presence of CCCP (30 μM) for 24 h and then subjected to immunoblot analysis. (d) Densitometric quantitation of EGFP fusion protein abundance in immunoblots similar to those in (c). Data are expressed relative to the corresponding control value (CCCP 0 h) and are means±s.d., from three independent experiments. **P<0.01 (Student’sttest). (e) MEFs stably expressing EGFP-Bcl-2(H235R) and FLAG-Parkin were incubated in the absence or presence of CCCP (30 μM) for 4 h, fixed, permeabilized and subjected to immunofluorescence analysis with antibodies to cytochromecand to FLAG (rabbit polyclonal). The fluorescence of EGFP-Bcl-2(H235R) was also monitored directly. Higher-magnification views of the boxed areas are shown in the right panels of each set. (f) Photoconversion assay with KikGR fusion proteins. Cells are exposed to UV (364 nm) and then treated with CCCP to induce mitophagy. Red signals represent preexisting protein, whereas green signals represent newly synthesized protein. (g) HeLa cells stably expressing FLAG-Parkin were transiently transfected with vectors for KikGR-FKBP38ΔN47 or KikGR-FKBP38ΔN47(N402K), exposed to UV, incubated in the absence or presence of CCCP (10 μM) for 4 h, and then monitored for red and green KikGR fluorescence. Scale bar (a,b,e,g), 10 μm. Full size image Figure 7: Basic residues in the CSS determine protein translocation during mitophagy. ( a ) MEFs stably expressing EGFP-FKBP38(N402K) and FLAG-Parkin were incubated in the absence or presence of CCCP (30 μM) for 4 h, fixed, permeabilized and subjected to immunofluorescence analysis with antibodies to cytochrome c and to FLAG (rabbit polyclonal). The fluorescence of EGFP-FKBP38(N402K) was also monitored directly. Higher-magnification views of the boxed areas are shown in the right panels of each set. ( b ) MEFs stably expressing EGFP-FKBP38(N402K), mCherry-FKBP38 and FLAG-Parkin were incubated in the absence or presence of CCCP (30 μM) for 4 h, fixed, permeabilized and subjected to immunofluorescence analysis with antibodies to FLAG (M2). The fluorescence of EGFP-FKBP38(N402K) and mCherry-FKBP38 was also monitored directly. ( c ) MEFs stably expressing FLAG-Parkin and either EGFP-FKBP38 or EGFP-FKBP38(N402K) were incubated in the absence or presence of CCCP (30 μM) for 24 h and then subjected to immunoblot analysis. ( d ) Densitometric quantitation of EGFP fusion protein abundance in immunoblots similar to those in ( c ). Data are expressed relative to the corresponding control value (CCCP 0 h) and are means±s.d., from three independent experiments. ** P <0.01 (Student’s t test). ( e ) MEFs stably expressing EGFP-Bcl-2(H235R) and FLAG-Parkin were incubated in the absence or presence of CCCP (30 μM) for 4 h, fixed, permeabilized and subjected to immunofluorescence analysis with antibodies to cytochrome c and to FLAG (rabbit polyclonal). The fluorescence of EGFP-Bcl-2(H235R) was also monitored directly. Higher-magnification views of the boxed areas are shown in the right panels of each set. ( f ) Photoconversion assay with KikGR fusion proteins. Cells are exposed to UV (364 nm) and then treated with CCCP to induce mitophagy. Red signals represent preexisting protein, whereas green signals represent newly synthesized protein. ( g ) HeLa cells stably expressing FLAG-Parkin were transiently transfected with vectors for KikGR-FKBP38ΔN47 or KikGR-FKBP38ΔN47(N402K), exposed to UV, incubated in the absence or presence of CCCP (10 μM) for 4 h, and then monitored for red and green KikGR fluorescence. Scale bar ( a , b , e , g ), 10 μm. Full size image In a converse approach, we also reduced the basicity of the CSS of Bcl-x L by generating the mutants Bcl-x L (R232S) and Bcl-x L (K233S), in which either arginine or lysine in the CSS was replaced with serine ( Fig. 6 ). The EGFP-tagged forms of these mutants localized to the mitochondria, but a small proportion of the mutant molecules underwent translocation on exposure of the cells to CCCP for 4 h ( Supplementary Fig. S10 ). We also tested the behaviour of Bcl-x L (ΔRK), in which both arginine and lysine had been removed from the COOH-terminus, leaving no basic amino acids in the CSS ( Fig. 6 ). EGFP-tagged Bcl-x L (ΔRK) localized to the ER in the absence or presence of CCCP, and it was therefore not degraded during mitophagy (data not shown). Together, these results thus suggested that a difference of only one amino acid in the CSS can determine the fate of mitochondrial proteins during mitophagy. Translocation is mediated by microtubule-dependent transport To confirm that FKBP38 detected at the ER after exposure of cells to CCCP is indeed transported from the mitochondria and does not represent newly synthesized protein, we took advantage of the photoconverting fluorescent protein Kikume Green-Red (KikGR), which emits green fluorescence that is converted to red after exposure to weak ultraviolet light [31] . Given that full-length FKBP38 tagged with KikGR tends to form aggregates in HeLa cells, we selected for our experiments KikGR-tagged FKBP38ΔN47, a mutant that lacks the 47 NH 2 -terminal residues and that shows a reduced tendency to aggregate when fused with KikGR. We confirmed that this deletion did not affect the behaviour of FKBP38 or FKBP38(N402K) during mitophagy ( Supplementary Fig. S11 ). We transfected HeLa cells with vectors encoding FLAG-Parkin and either KikGR-FKBP38ΔN47 or KikGR-FKBP38ΔN47(N402K), the latter of which contains a point mutation to prevent escape from the mitochondria. The cells were then exposed to UV (364 nm) in order to convert the green fluorescence emitted by mitochondrial KikGR-FKBP38ΔN47 or its point mutant to red, after which they were treated with CCCP to induce mitophagy ( Fig. 7f ). Protein molecules that are newly synthesized after UV irradiation would thus be expected to emit green fluorescence and therefore be distinguishable from those localized to the mitochondria before CCCP treatment. As expected, KikGR-FKBP38ΔN47(N402K) red signals had become concentrated in the perinuclear region as a result of mitophagy by 4 h after the onset of CCCP treatment, whereas KikGR-FKBP38ΔN47 red signals had translocated from the mitochondria to the ER ( Fig. 7g ; Supplementary Fig. S12 ; Supplementary Movie 2 ). We also examined the effects of inhibiting protein synthesis with cycloheximide (CHX) in NIH 3T3 cells. Given that CHX inhibited the progression of mitophagy ( Supplementary Fig. S13a ), we exposed cells to CCCP for 2 h before CHX treatment. Under this condition, immunofluorescence analysis revealed that FKBP38 signals became diffusely dispersed and did not colocalize with cytochrome c ( Supplementary Fig. S13b ). Immunoblot analysis of subcellular fractions revealed that FKBP38 and Bcl-2 appeared in the ER fraction in response to such treatment with CCCP and CHX ( Supplementary Fig. S13c ). Collectively, these results confirmed that FKBP38 localized at the ER after CCCP treatment is not a newly synthesized protein but rather a protein transported from the mitochondria. We next examined whether FKBP38 translocation from damaged mitochondria to the ER depends on tethering between these organelles mediated by Mitofusin 2 (Mfn2) [32] . Immunofluorescence signals for FKBP38 showed a diffuse distribution suggestive of ER localization and were not colocalized with those for cytochrome c in both Mfn2 +/+ and Mfn2 −/− MEFs treated with CCCP for 4 h ( Fig. 8a ). Immunoblot analysis also revealed that the abundance of cytochrome c decreased, with the protein eventually disappearing by 24 h, after the onset of CCCP exposure in both Mfn2 +/+ and Mfn2 −/− MEFs, whereas the amounts of FKBP38 and Bcl-2 had not decreased at this time in the MEFs of either genotype ( Fig. 8b ). These results thus suggested that the translocation of FKBP38 and Bcl-2 during mitophagy is not dependent on Mfn2-mediated tethering between the mitochondria and the ER. 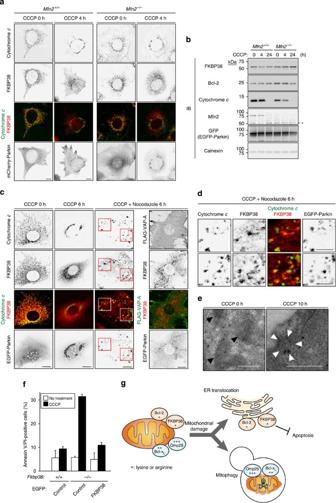Figure 8: FKBP38 translocation to the ER is mediated by microtubule-dependent transport. (a) Wild-type (Mfn2+/+) andMfn2knockout (Mfn2–/–) MEFs stably expressing mCherry-Parkin were incubated in the absence or presence of CCCP (30 μM) for 4 h, fixed, permeabilized and subjected to immunofluorescence analysis with antibodies to FKBP38 and to cytochromec. The fluorescence of mCherry-Parkin was also monitored directly. (b) MEFs as inabut expressing EGFP-Parkin were treated with CCCP (30 μM) for the indicated times and then subjected to immunoblot analysis. The asterisk indicates a nonspecific band. (c) Wild-type MEFs stably expressing EGFP-Parkin and FLAG-VAP-A were incubated in the absence or presence of CCCP (30 μM) or nocodazole (10 μM) for 6 h as indicated, fixed, permeabilized and subjected to immunofluorescence analysis with antibodies to cytochromec, to FLAG and to FKBP38. The fluorescence of EGFP-Parkin was also monitored directly. (d) Higher-magnification views of the boxed areas in (c,e). Wild-type MEFs stably expressing FLAG-Parkin and EGFP-FKBP38 were incubated in the absence or presence of CCCP (30 μM) for 10 h and then subjected to immuno-electron microscopic analysis with antibodies to GFP. Black arrowheads indicate the mitochondria. White arrowheads indicate small vesicle. (f) Wild-type (Fkbp38+/+) andFkbp38knockout (Fkbp38−/−) MEFs stably expressing FLAG-Parkin and either EGFP or EGFP-FKBP38 were incubated in the absence or presence of CCCP (30 μM) for 24 h and then stained with allophycocyanin (APC)-labelled annexin V and propidium iodide (PI) for flow cytometric analysis of the percentage of apoptotic cells (annexin V+and PI+cells). Data are means±s.d., from three independent experiments. (g) Model for FKBP38 and Bcl-2 translocation from the mitochondria. Damaged mitochondria accumulate PINK1 and recruit Parkin. FKBP38 and Bcl-2 then translocate from the damaged mitochondria to the ER in order to escape degradation during mitophagy. Scale bars (a,c,d), 10 μm; (e), 500 nm. Figure 8: FKBP38 translocation to the ER is mediated by microtubule-dependent transport. ( a ) Wild-type ( Mfn2 +/+ ) and Mfn2 knockout ( Mfn2 –/– ) MEFs stably expressing mCherry-Parkin were incubated in the absence or presence of CCCP (30 μM) for 4 h, fixed, permeabilized and subjected to immunofluorescence analysis with antibodies to FKBP38 and to cytochrome c . The fluorescence of mCherry-Parkin was also monitored directly. ( b ) MEFs as in a but expressing EGFP-Parkin were treated with CCCP (30 μM) for the indicated times and then subjected to immunoblot analysis. The asterisk indicates a nonspecific band. ( c ) Wild-type MEFs stably expressing EGFP-Parkin and FLAG-VAP-A were incubated in the absence or presence of CCCP (30 μM) or nocodazole (10 μM) for 6 h as indicated, fixed, permeabilized and subjected to immunofluorescence analysis with antibodies to cytochrome c , to FLAG and to FKBP38. The fluorescence of EGFP-Parkin was also monitored directly. ( d ) Higher-magnification views of the boxed areas in ( c , e ). Wild-type MEFs stably expressing FLAG-Parkin and EGFP-FKBP38 were incubated in the absence or presence of CCCP (30 μM) for 10 h and then subjected to immuno-electron microscopic analysis with antibodies to GFP. Black arrowheads indicate the mitochondria. White arrowheads indicate small vesicle. ( f ) Wild-type ( Fkbp38 +/+ ) and Fkbp38 knockout ( Fkbp38 −/− ) MEFs stably expressing FLAG-Parkin and either EGFP or EGFP-FKBP38 were incubated in the absence or presence of CCCP (30 μM) for 24 h and then stained with allophycocyanin (APC)-labelled annexin V and propidium iodide (PI) for flow cytometric analysis of the percentage of apoptotic cells (annexin V + and PI + cells). Data are means±s.d., from three independent experiments. ( g ) Model for FKBP38 and Bcl-2 translocation from the mitochondria. Damaged mitochondria accumulate PINK1 and recruit Parkin. FKBP38 and Bcl-2 then translocate from the damaged mitochondria to the ER in order to escape degradation during mitophagy. Scale bars ( a , c , d ), 10 μm; ( e ), 500 nm. Full size image To determine whether FKBP38 translocation from damaged mitochondria to the ER is mediated by the microtubule-dependent transport system, we treated MEFs expressing EGFP-Parkin with both CCCP and the microtubule-destabilizing agent nocodazole for 6 h. Although nocodazole affected the aggregation of damaged mitochondria around the nuclear membrane [33] , signals for FKBP38 remained colocalized with those for cytochrome c in the presence of this agent ( Fig. 8c ), suggesting that nocodazole inhibited FKBP38 translocation. Immuno-electron microscopy revealed that signals for EGFP-FKBP38 that had initially localized at the mitochondria were associated with small vesicular structures at 10 h after the onset of CCCP exposure ( Fig. 8e ). These results thus indicated that FKBP38 translocation from damaged mitochondria to the ER is mediated by microtubule-dependent vesicular transport. Finally, to investigate the physiological relevance of the coordinated translocation of FKBP38 and Bcl-2, we examined the sensitivity of Fkbp38 +/+ and Fkbp38 −/− MEFs to apoptosis during mitophagy. FKBP38 is not necessary for the induction of mitophagy itself ( Supplementary Fig. S14a ). The sensitivity to apoptosis during CCCP exposure, however, was markedly increased for Fkbp38 −/− MEFs compared with the control cells, and forced expression of EGFP-FKBP38 in the FKBP38-null cells reversed this phenotype ( Fig. 8f ; Supplementary Fig. S14b–d ). These results thus suggested that FKBP38 translocation to the ER is essential for suppression of unwanted apoptosis during mitophagy. We have found that not all mitochondrial proteins are eliminated during the massive protein degradation associated with mitophagy. Rather, certain mitochondrial outer membrane proteins, including FKBP38 and Bcl-2, escape from the mitochondria to the ER in order to avoid degradation ( Fig. 8g ). This phenomenon is highly selective, given that structurally and functionally similar proteins such as Bcl-2 and Bcl-x L show different fates. The molecular basis for this selectivity appears to be the basicity of the CSS, with a difference of only one amino acid being sufficient to confer a different fate, although this conclusion remains to be verified by examination of additional proteins. Most mitochondrial proteins are synthesized as cytosolic precursors and contain a mitochondrial targeting signal at their NH 2 -terminus that facilitates transport into the mitochondria through the TOM complex [34] . However, some mitochondrial outer membrane proteins—including FKBP38, Bcl-2, Bcl-x L and Omp25—contain a mitochondrial targeting signal known as a ‘tail anchor’ at their COOH-terminus [35] . Such tail-anchored proteins are thought to be integrated into the lipid bilayer of the mitochondrial outer membrane by the ‘unassisted pathway’ [36] , [37] . The mechanism underlying mitochondrial targeting by the tail anchor was examined in a study that focused on differences in amino-acid sequence between the CSS of Bcl-2 and that of Bcl-x L [30] . Mutagenesis revealed that the basicity of the CSS determines the mitochondrial targeting of these proteins. However, protein evacuation during mitophagy and the role of mitochondrial targeting sequences in such translocation have not been described. We now show that the CSS has a pivotal role not only in mitochondrial targeting but also in protein escape from the mitochondria during mitophagy. Basic amino acids in the CSS might serve as a latch to retain tail-anchored proteins at the mitochondrial outer membrane. Bcl-x L , which contains two basic amino acids in its CSS, might thus be stably anchored to the membrane, whereas Bcl-2, which contains only one basic amino acid in its CSS, might shuttle between the mitochondria and the ER and be readily detached from the mitochondrial outer membrane. FKBP38 functions to recruit Bcl-2 to the mitochondria, and it also evacuates from the mitochondria during mitophagy. The coordinated translocation of FKBP38 and Bcl-2 might control the sensitivity of cells to apoptosis. Contact between the mitochondria and the ER has a role in mitochondrial division [38] , [39] . In yeast, ER–mitochondrial communication is thought to occur through direct contact between the membranes of these organelles, which gives rise to the formation of an ER–mitochondrial encounter structure [40] , [41] . In mammals, a structure termed MAM (mitochondria-associated ER membrane) has been shown to contribute to the regulation of signal transduction, biogenesis, cell death and lipid metabolism [42] , [43] , [44] . Physical tethers are also thought to be important for the stable positioning of the mitochondria for efficient energy utilization at specific locations within the cell, such as in axons and dendrites of neurons [39] , [45] . However, the effects of nocodazole treatment in the present study indicate that microtubule polymerization is required for the translocation of FKBP38 from the mitochondria to the ER. Vesicle transport occurs between various organelles, with such communication having recently been shown to take place between the mitochondria and both peroxisomes and lysosomes [46] , [47] . Small vesicles might thus be generated as a consequence of mitochondrial membrane damage and then be transported to the ER by the microtubule-dependent trafficking system. The regulation of this process as well as the possibility of opposite transport from the ER to the mitochondria remains to be investigated. Construction of plasmids Construction of vectors encoding human or mouse FKBP38, human Bcl-2, mouse Bcl-x L and human VAP-A was described previously [21] , [25] . Human Parkin cDNA was kindly provided by T. Kanki (Kyushu University), mouse Omp25 cDNA by K. Mihara (Kyushu University) and rat LC3 cDNA by N. Mizushima (Tokyo Medical and Dental University). Complementary DNAs were subcloned into the pEGFP vector (Clontech, Mountain View, CA), humanized-codon monomeric KikGR vector (MBL, Nagoya, Japan) or pMX-puro vector. Cell culture and transfection Plat-E, HeLa, HEK293T and SH-SY5Y cells were maintained in Dulbecco’s modified Eagle’s medium (DMEM) supplemented with 10% fetal bovine serum (Invitrogen, Carlsbad, CA); the medium for Plat-E cells was also supplemented with blasticidin (10 μg ml −1 ). NIH 3T3 cells were maintained in DMEM supplemented with 10% calf serum (Invitrogen). Primary MEFs were prepared as described previously [48] , [49] ; nonsenescent MEFs were used for all experiments. Mfn2 +/+ and Mfn2 −/− MEFs were kindly provided by T. Koshiba and D.C. Chan (California Institute of Technology). Retroviral infection was performed as previously described [50] . For lentiviral infection, a DNA fragment encoding a stem-loop-type short hairpin RNA specific for human Parkin mRNA (5′-GGAAGTCCAGCAGGTAGATCA-3′) was synthesized, attached to the U6 promoter and subcloned into the vector pCSII (kindly provided by H. Miyoshi, RIKEN), and lentiviruses were produced by HEK293T cells. The cells were transfected using the calcium phosphate method for 24 h at 37 °C, after which the medium was replaced and the cells were incubated for an additional 24 h for collection of virus-containing culture supernatants. SH-SY5Y cells were plated in six-well plates 24 h before infection. Other cell types were transfected with expression vectors with the use of FuGENE HD. For induction of mitochondrial depolarization, HeLa and SH-SY5Y cells were treated with 10 μM CCCP, whereas MEFs and NIH 3T3 cells were treated with 30 μM CCCP. For amino-acid deprivation, cells were washed with PBS and incubated in amino-acid-free DMEM without serum. Antibodies For immunoblot analysis and immunofluorescence staining, rabbit polyclonal antibodies specific for FKBP38 (FK38N1) were generated in response to a His 6 -tagged recombinant protein comprising the NH 2 -terminal half of FKBP38 that was expressed in and purified from Escherichia coli [21] . Rabbit polyclonal antibodies to LC3 were kindly provided by N. Mizushima, and those to TOM40 were kindly provided by K. Mihara. Mouse monoclonal antibodies to Bcl-2 (610538), to cytochrome c (556432, 556433), to Tim23 (611222), to BiP/GRP78 (610978) and to HSP90 (610419) were obtained from BD Biosciences (San Jose, CA), those to HA epitope (HA-11) were from Research Diagnostics (Flanders, NJ) and those to multiubiquitin (FK2) were from Nippon Bio Test Laboratory (Tokyo, Japan); rabbit polyclonal antibodies to calnexin were from Stressgen (Victoria, British Columbia, Canada), those to PINK1 (BC100-494) were from Novus Biologicals (Littleton, CO), and those to GFP (sc-8334), to TOM20 (sc-11415), to Mfn2 (sc-100560) and to Bcl-x S/L (S-18) (sc-634) were from Santa Cruz Biotechnology (Santa Cruz, CA); rabbit monoclonal antibodies to p70 S6 kinase (49D7) and to Thr 389 -phosphorylated p70 S6 kinase (108D2) were from Cell Signaling (Beverly, MA); rabbit polyclonal antibodies to GFP (ab6556) were also obtained from Abcam (Cambridge, UK); antibodies to FLAG (mouse monoclonal M2 and rabbit polyclonal) and mouse monoclonal antibodies to Parkin (PRK8) were from Sigma (St Louis, MO). Alexa Fluor 488-, Alexa Fluor 546- or Alexa Fluor 633-conjugated goat antibodies to mouse or rabbit immunoglobulin G as well as streptavidin-Alexa Fluor 546 were obtained from Molecular Probes (Eugene, OR). Colloidal gold (10 nm)-conjugated goat antibodies to rabbit immunoglobulin G were obtained from EY labs (San Mateo, CA). Chemicals Stock solutions of CCCP, Bafilomycin A1 and CHX (Wako, Osaka, Japan), of paraquat (Santa Cruz Biotechnology), of lactacystin (Peptide Institute, Osaka, Japan), and of nocodazole (Sigma) were prepared in dimethyl sulphoxide or water. Immunoblot analysis Cells were lysed in a solution containing 40 mM HEPES-NaOH (pH 7.6), 150 mM NaCl, 10% glycerol, 0.5% Triton X-100, 1 mM Na 3 VO 4 , 25 mM NaF, 1 mM phenylmethylsulphonyl fluoride, aprotinin (10 μg ml −1 ) and leupeptin (10 μg ml −1 ). The lysate was subjected to immunoblot analysis as previously described [50] . Full-length scans of key immunoblots shown in the main figures are presented in Supplementary Figure S15 . Immunofluorescence staining MEFs, SH-SY5Y cells or HeLa cells grown on glass coverslips were washed with PBS, fixed for 10 min at room temperature with 4% formaldehyde in PBS, washed again, and then incubated for 2 h at room temperature with primary antibodies in PBS containing 0.1% bovine serum albumin and 0.1% saponin. After washing, the cells were incubated for 30 min at room temperature with Alexa Fluor-labelled goat secondary antibodies at a dilution of 1:2,000 in PBS containing 0.1% bovine serum albumin and 0.1% saponin. They were washed again and then covered with a drop of GEL/MOUNT (Biomeda, Foster City, CA) for examination with a confocal fluorescence microscope (LSM510 META, Carl Zeiss) equipped with an X63/1.4 oil-immersion objective. For staining of the mitochondria, cells were incubated for 20 min with 100 nM MitoTracker (Molecular Probes) before fixation. Cell fractionation NIH 3T3 cells were suspended in isolation buffer (250 mM mannitol, 1 mM EGTA-Tris and 10 mM HEPES-NaOH, pH 7.5) and disrupted by dounce homogenization. The homogenate was centrifuged at 800 g for 10 min at 4 °C, and the resulting supernatant was further centrifuged at 8,000 g for 10 min at 4 °C. The new pellet (crude mitochondrial fraction) was collected, and the supernatant was centrifuged further at 100,000 g for 30 min at 4 °C. The resulting pellet (light membrane fraction) and supernatant (cytosolic fraction) were collected. The crude mitochondrial fraction was layered on a solution of 30% Percoll (GE Healthcare) in isolation buffer and centrifuged at 100,000 g for 30 min at 4 °C. The resulting mitochondrial and ER bands were isolated, washed free of Percoll and resuspended in isolation buffer. Photoconversion analysis Photoconversion analysis of cells expressing KikGR-labelled proteins was performed with 10–15 bleach cycles with a 364-nm UV laser and with the use of the photobleach function of the LSM510 META microscope. Detection of apoptosis For detection of apoptosis, cells were washed twice with ice-cold PBS and then stained simultaneously with allophycocyanin-conjugated annexin V and propidium iodide (PI) (both from BD Biosciences) in a solution containing 10 mM HEPES-NaOH (pH 7.4), 140 mM NaCl and 2.5 mM CaCl 2 for 20 min on ice and in the dark. Within the next hour, the cells were analysed with a FACS Calibur flow cytometer and Cell Quest software (Becton Dickinson, San Jose, CA) and the total number of apoptotic cells (annexin V + and PI + cells) was determined. For the TUNEL (terminal deoxynucleotidyl transferase-mediated dUTP-biotin nick end labelling) assay, MEFs grown on glass coverslips were washed with PBS, fixed for 30 min at 4 °C with 70% ethanol in PBS, washed again and then incubated for 1 h at 37 °C with a reaction mixture containing terminal deoxynucleotidyl transferase (Invitrogen) and biotinylated dUTP (Roche Applied Science). Labelled DNA was visualized with a confocal fluorescence microscope (LSM510 META). MEFs first treated with DNase (Wako) were used as a positive control, whereas the transferase was omitted from the reaction mixture as a negative control. Time-lapse imaging HeLa cells expressing mCherry-Parkin and EGFP-tagged forms of FKBP38, Omp25 or Bcl-2 were plated on a glass-bottom dish and then treated with 10 μM CCCP. Images of the cells examined with a fluorescence microscope (IX81, Olympus) were collected every 2 min for 6 h. HeLa cells expressing FLAG-Parkin and KikGR-labelled forms of FKBP38ΔN47 or FKBP38ΔN47(N402K) were plated on a glass-bottom dish, exposed to UV light and then treated with 10 μM CCCP. Images of the cells examined with the IX81 fluorescence microscope were collected every 30 min for 4 h. Immuno-electron microscopy MEFs were fixed with 4% paraformaldehyde and 0.4% glutaraldehyde in 0.1 M cacodylate buffer (pH 7.4) for 1 h on ice, treated with 0.05 M NH 4 Cl in PBS, dehydrated in a graded series of ethanol solutions, embedded in LR white resin (medical grade; Electron Microscopy Sciences, Fort Washington, PA), exposed to UV radiation for 3 days at −20 °C and then incubated for 24 h at 65 °C. Pale gold ultrathin sections were collected on Formvar-carbon-coated nickel grids, which were then exposed to PBS containing 3% bovine serum albumin before incubation for 24 h at 4 °C with primary antibodies in PBS containing 3% bovine serum albumin. The grids were washed, incubated for 1 h at 37 °C with colloidal gold (10 nm)-conjugated goat secondary antibodies at a dilution of 1:50 in PBS, exposed to 0.5% osmium tetroxide and treated with 2% uranyl acetate to confer a light contrast. The sections were examined with a Tecnai-20 transmission electron microscope (FEI, Hillsboro, OR), and images were collected with an Eagle 2k HR digital camera (FEI). Statistical analysis Data are presented as means±s.d., and were compared using Student’s t -test. A P -value of <0.05 was considered statistically significant. How to cite this article : Saita, S. et al . Selective escape of proteins from the mitochondria during mitophagy. Nat. Commun. 4:1410 doi: 10.1038/ncomms2400 (2013).